Environmental variability promotes plant invasion Global environmental change not only entails changes in mean environmental conditions but also in their variability. Changes in climate variability are often associated with altered disturbance regimes and temporal patterns of resource availability. Here we show that increased variability of soil nutrients strongly promotes another key process of global change, plant invasion. In experimental plant communities, the success of one of the world's most invasive plants, Japanese knotweed, is two- to four-fold increased if extra nutrients are not supplied uniformly, but in a single large pulse, or in multiple pulses of different magnitudes. The superior ability to take advantage of variable environments may be a key mechanism of knotweed dominance, and possibly many other plant invaders. Our study demonstrates that increased nutrient variability can promote plant invasion, and that changes in environmental variability may interact with other global change processes and thereby substantially accelerate ecological change. Environmental change can come in two forms: a change in mean conditions [1] , or a change in environmental variability, for example, when the degree of stochasticity of environments increases or extreme events become more frequent [2] , [3] , [4] . We know that both kinds of change can strongly impact natural ecosystems [5] , [6] , [7] , but as previous ecological research typically focused on changes in means, we still have a much more limited understanding of the ecological consequences of changes in variability, and their potential interactions with other drivers of change [8] , [9] . In particular, there is a dearth of experimental studies that truly tested for the consequences of changes in variability per se by explicitly manipulating environmental variability, while holding constant environmental means. From an ecological perspective, changes in environmental variability impose a different set of challenges to organisms than changes in environmental means [8] . Among others, greater environmental variability is often associated with increased disturbance and, ultimately, variability of resource supply. This is obvious in the case of extreme events such as drought or flooding, but it may also be true for more subtle changes of environmental variability. For instance, nutrient uptake by plants critically depends on soil moisture, and therefore increased variability of precipitation is inevitably linked to the variability of nutrient supply [10] , [11] . Changes in environmental variability could significantly interact with other global change processes, such as biological invasions. Several years ago, Davis et al . [12] proposed that habitats with a high variability of resource availability will generally be more easily invaded than habitats with less variable resource conditions. However, although this theory of fluctuating resource availability has become a cornerstone of invasion biology, clear-cut experimental tests of its predictions are still rare. To test the potential effects of increased resource variability on plant invasions, we conducted an ecological experiment with one of the world’s most invasive plants, Japanese knotweed, and show that its invasion success is strongly increased when nutrients are supplied in a non-uniform manner. Ecological experiment We conducted an experiment in which Japanese knotweed s.l. ( Fallopia spp. ; Fig. 1 ) invaded experimental communities of native plants ( Fig. 1b ) under five different scenarios of nutrient supply ( Fig. 2a ): (i) constant low or (ii) constant high supply, (iii) gradual increase, (iv) a single large nutrient pulse or (v) multiple pulses of different magnitudes. All experimental treatments but the first one received the same total amount of resources. Compared with (ii), scenarios (iii)–(v) thus constituted scenarios with increased environmental variability. 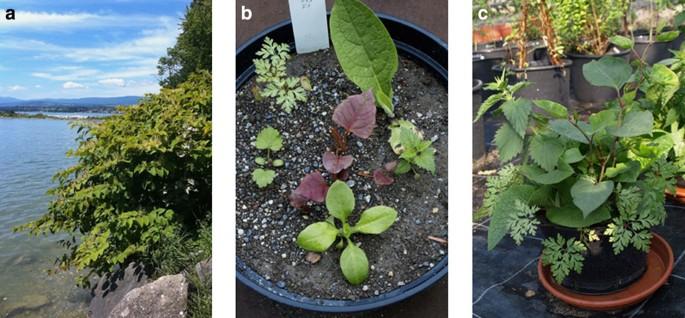Figure 1: Invasive knotweed in an invaded habitat and in our experiment. (a) An invasive population at the shore of Lake Geneva, Switzerland. (b) An experimental community, shortly after planting, with knotweed in the centre, surrounded by five native species. (c) An established community at the time of peak growth. Figure 1: Invasive knotweed in an invaded habitat and in our experiment. ( a ) An invasive population at the shore of Lake Geneva, Switzerland. ( b ) An experimental community, shortly after planting, with knotweed in the centre, surrounded by five native species. ( c ) An established community at the time of peak growth. 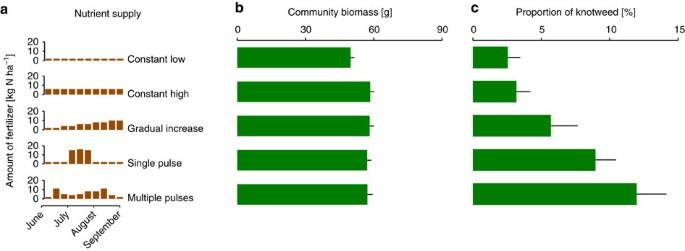Figure 2: Invasion success of exotic knotweedFallopiaspp. in experimental communities of native European plants, under five different scenarios of nutrient supply. (a) Temporal patterns of nutrient supply, with the amounts of nitrogen applied at each of ten application times. The total amount of nitrogen is constant in all but the first. (b) Total biomass of the plant community. (c) Invasion success of knotweed, measured as the percentage of community biomass it represented. The bars in (b,c) represent means plus s.e. of the means. Full size image Figure 2: Invasion success of exotic knotweed Fallopia spp. in experimental communities of native European plants, under five different scenarios of nutrient supply. ( a ) Temporal patterns of nutrient supply, with the amounts of nitrogen applied at each of ten application times. The total amount of nitrogen is constant in all but the first. ( b ) Total biomass of the plant community. ( c ) Invasion success of knotweed, measured as the percentage of community biomass it represented. The bars in ( b , c ) represent means plus s.e. of the means. Full size image We found that changes in resource variability had no effect on the total biomass of plant communities ( F 3,118 =0.08, P =0.97; Fig. 2b ), but they strongly shifted the competitive balance between knotweed and native plants towards the invader ( F 3,118 =10.69, P <0.001; Fig. 2c ). If resources were gradually increasing over time rather than supplied at a constant rate, the success of knotweed more than doubled, and it even tripled if resources were supplied in a single extreme event. The greatest increase of knotweed success occurred where resources were supplied unpredictably through multiple pulses of varying magnitudes ( Fig. 2c ). One important conclusion from our study is that environmental variability can strongly promote the invasion of knotweed, and possibly of many other invasive plants. In their introduced range, invasive knotweeds are most dominant, and cause great damage, along rivers where periodic floods create disturbance and nutrient pulses. A key mechanism explaining this dominance might be the knotweeds’ superior ability to capitalize on periods of highresource availability, presumably because they can respond quicker to nutrient pulses, or have a higher maximum growth rate, than native plant species. A high growth rate and the ability to rapidly exploit high-resource conditions are widely recognized as fundamental plant strategies [13] , and a potential determinant of invasion success [14] . Recent meta-analyses have shown that these characteristics are indeed overrepresented among successful plant invaders [15] , [16] . Given that disturbed, nutrient-rich habitats are almost universally the most invaded ones [17] , this strongly suggests that environmental variability is a key driver of many plant invasions, and increased variability will promote the further spread of invasive species. Our study provides support for the fluctuating resource availability hypothesis [12] , and it confirms the results of the handful of studies, which so far explicitly tested it [18] , [19] . Future studies should more frequently test the effects of changes in resource variability independently of changes in resource means. They should in particular address the generality of the observed effects across different resources and invasive species, as well as different timings and temporal patterns of resource pulses, and they should attempt to identify the specific mechanisms—for example, speed of response versus maximum growth rate—that make plants successful under these conditions. The second, more general, conclusion from our study is that an increase in variability can be a strong driver of ecological change in itself, and that, when studying this driver, it can be very informative to go beyond the effects of climate extremes, and to incorporate other environmental factors, other forms of variability, and interactions with other drivers of change. If increases in environmental variability will indeed, as predicted by models [20] , [21] , intensify in the future, and this will, as in our study, feed back on other drivers and thereby accelerate ecological change, then future biodiversity changes may so far have been considerably underestimated, particularly in those areas for which the greatest increases of environmental variability are predicted. Experiment We set up an experiment in which artificial communities of native European plants were invaded by exotic knotweed. We attempted to make this experiment as ecologically realistic as possible—by using local, natural substrates and plant materials, and by working with communities rather than individual native plants—while maintaining experimental control over the total amount and temporal patterns of nutrient availability. For the native communities, we used five forbs ( Geranium robertianum, Geum urbanum, Silene dioica, Symphytum officinale, Urtica dioica ) that are common in the habitats invaded by knotweed. We used seed material from a regional supplier of wild-collected seeds (Rieger-Hofmann GmbH, Blaufelden-Raboldshausen, Germany). As invaders, we used the two most invasive knotweed taxa Fallopia japonica and the hybrid Fallopia × bohemica . We used rhizomes that had been collected in invasive populations in Germany and Switzerland, and propagated in a common garden for several years. In May 2010, we filled 150 4 l pots with a 1:1 mixture of sand and field soil (RICOTER Erdaufbereitung AG, Aarberg, Switzerland). Into each pot we planted one seedling from each of the native species, plus one knotweed rhizome (8–10 cm, two nodes). In half of the pots, we planted rhizomes of F. japonica , in the other half Fallopia × bohemica . The rhizomes were buried 5 cm deep in the centre of the pot, and the natives planted in a circle around it ( Fig. 1b ). Rhizomes and seedlings were randomly assigned to pots, and the planting order of natives was randomized. The experiment was set up in a large greenhouse, where the sides had been removed, essentially under a glass roof, in Muri b. Bern, Switzerland. One month after the setup, 15 pots per knotweed taxon were randomly assigned to each of five nutrient supply scenarios. We used liquid NPK (7:5:6) fertilizer, applied at 10 different time points, every 10 days, to create five different temporal patterns of nutrient supply ( Fig. 2a ): (i) constant low (20 kg ha −1 ), (ii) constant high (60 kg ha −1 ), (iii) gradual increase, (iv) single large pulse or (v) multiple pulses of different magnitudes. The same total amounts of nutrients were added in treatments (ii) to (v), only with different temporal patterns of supply. The large pulse started 2 months after experimental setup, at a time when all plants were growing vigorously. For the multiple pulses, one random temporal pattern of extra nutrient supply was used for all replicates of the treatment. During the experiment, the pots were watered as needed, and all pots received the same amounts of water. In September 2010, we cut the above-ground biomass of all plants, separated it by species, dried it at 80 °C until constant weight and weighed it. Data analysis For each pot, we calculated total community biomass by summing up the biomasses of all species, and as a measure of invasion success we calculated the percentage of total biomass that was represented by knotweed. The data were analyzed with general linear models that initially included nutrient level (low versus high), variability (the four scenarios at high nutrient level) nested within nutrient level, Fallopia taxon, and their interactions, as fixed effects. However, as there never were any statistically significant differences between the Fallopia taxa, we dropped this factor, and its interactions, from the final analyses. The percentage data were arcsin square-root transformed before analyses. For the analyses we only used the 123 pots where Fallopia had resprouted (shoot appearance above ground) during the experiment (82% of the pots; no differences of resprouting between taxa or treatments). How to cite this article: Parepa, M. et al . Environmental variability promotes plant invasion. Nat. Commun. 4:1604 doi: 10.1038/ncomms2632 (2013).